Diversity-oriented synthesis ofLycopodiumalkaloids inspired by the hidden functional group pairing pattern Natural products continue to provide a rich source of inspiration for both chemists and biologists. The efficient synthesis of bioactive natural products or natural product-like molecules has offered tremendous opportunities for complex biological processes exploration and drug discovery. However, because natural products usually contain numerous stereogenic centres and polycyclic ring systems, significant synthetic challenges remain. Here we employ the build/couple/pair strategy that is frequently used in diversity-oriented synthesis to obtain skeletally diverse compounds with complexities comparable to natural products. Inspired by the functional group pairing patterns hidden in Lycopodium alkaloids, we efficiently and in parallel construct four natural products, (+)-Serratezomine A, (−)-Serratinine, (+)-8α-Hydroxyfawcettimine and (−)-Lycoposerramine-U, as well as six different unnatural scaffolds, following the advanced build/couple/pair algorithm. This newly developed strategy is expected to be applied to the efficient synthesis of other complex natural products possessing functional group pairing patterns as well as skeletally diverse natural product-like molecules. It is accepted that natural products have been the most productive source of leads in drug development [1] . The majority of natural products have complex structures with abundant stereochemistry, as well as various ring systems and functional groups, providing a multitude of three-dimensional frameworks that occupy a different and wider chemical space in comparison with unnatural compounds [2] , [3] . As reported by Hert et al. [4] , 83% of the core ring scaffolds from natural products are not found in commercially available molecules and screening libraries [3] . In fact, when they are included in a screening library, natural products and their synthetic analogues may improve the hit rate. Nevertheless, to meet the urgent need for natural products or skeletally diverse natural product-like compounds, chemists are confronted with significant synthetic challenges in terms of efficiently generating structural complexity. Classically, there are three major strategies to access diverse natural products or analogues ( Fig. 1a ): divergent total synthesis ( I ), functional group diversification ( II ) and skeletal diversification ( III ) of natural product(s). Divergent total synthesis ( I ) is a widely applied approach for constructing several members of a family of related natural products, but it is rarely utilized for further diversification of a polycyclic scaffold [5] , [6] , [7] , [8] . Functional group diversification ( II ) of natural product is usually aimed at constructing a library of analogues or derivatives for structure–activity relationship studies and subsequent target identification. A remarkable C−H amination approach was disclosed recently, which demonstrated an excellent example of direct functional group diversification of natural product for target identification [9] . Biology-oriented synthesis was also an excellent approach to construct focused library of natural product-like molecules [10] . In addition, several elegant examples of producing complex and skeletally diverse molecules directly from readily available natural products to achieve skeletal diversification ( III ) were also reported [11] , [12] , [13] . Moreover, a number of remarkable approaches have been utilized to realize both I and II (refs 14 , 15 ), which efficiently provided complex natural products and their derivatives in parallel. Although, biosynthesis has offered a lot of inspirations for natural product total synthesis as well as skeletal diversification [16] , [17] , [18] , [19] , it is challenging to devise a unified strategy to furnish natural products ( I ) and skeletally diverse natural product-like molecules ( III ) concurrently all starting from simple building blocks. 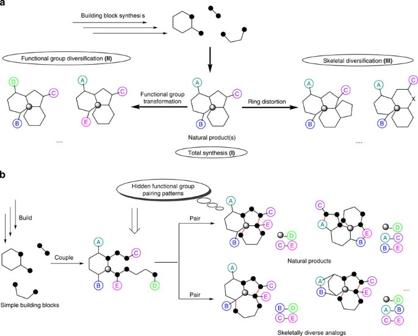Figure 1: Comparison of the classical strategies with the FGPPs inspired B/C/P strategy. (a) Classical strategies for the total syntheses as well as functional group and skeletal diversifications of natural products. (b) In our strategy, the hidden FGPPs of a class of natural products are first identified, and then a B/C/P process is designed to synthesize skeletally diverse analogues and natural products in parallel via different functional group pairing pathways. Circled letters A–E represent different functional groups, and the grey ball represents an active carbon center. The bond formations from hidden FGPPs are highlighted in red. Figure 1: Comparison of the classical strategies with the FGPPs inspired B/C/P strategy. ( a ) Classical strategies for the total syntheses as well as functional group and skeletal diversifications of natural products. ( b ) In our strategy, the hidden FGPPs of a class of natural products are first identified, and then a B/C/P process is designed to synthesize skeletally diverse analogues and natural products in parallel via different functional group pairing pathways. Circled letters A–E represent different functional groups, and the grey ball represents an active carbon center. The bond formations from hidden FGPPs are highlighted in red. Full size image In contrast, diversity-oriented synthesis (DOS) focuses on the efficient preparation of skeletally and stereochemically diverse molecules that will be further subjected to biological evaluations for drug discovery or chemical biology [20] , [21] , [22] . Among the strategies for DOS, the build/couple/pair (B/C/P) algorithm [23] is the most widely utilized. In this strategy, a collection of compounds with highly diverse scaffolds are generated via functional group pairing [24] reactions (the pair phase) using precursors bearing suitable functional groups that have been generated by coupling chiral building blocks (the couple phase) that are pre-synthesized in the build phase. As an improvement, Park [25] , [26] recently initiated a privileged substructure-based DOS strategy to generate skeletal diversity of natural product-like and drug-like molecules with high biological relevance. Although DOS has proven to be a successful strategy for the rapid access to chemical libraries of natural product-like three-dimensional molecular architectures from simple starting materials [27] , [28] , [29] , [30] , [31] , [32] , it was rarely applied to natural product total synthesis in parallel with skeletal diversification. Herein, we introduce a novel approach using DOS for the concise construction of both natural products and their analogues possessing diverse, highly complex skeletons in parallel. Typically, natural products have various functional groups that ‘pair’ together in different patterns (connecting via C−C, C−N, C−O or other bonds) [33] , [34] . In our strategy, complex molecules are synthesized by the following steps that take advantage of the B/C/P algorithm ( Fig. 1b ): (1) identifying the hidden functional group pairing patterns (FGPPs) in natural products and then ‘depairing’ them to afford a densely functionalized precursor; (2) performing reactions to provide this precursor through B/C phases; and (3) exploring a variety of functional group pairing reactions sequentially to afford the natural products and distinct natural product-like scaffolds in parallel. This approach is expected to be complementary to the current standard DOS strategy and should facilitate the synthesis and diversification of natural products in a highly efficient manner due to the characteristics of concurrent branch points. Design of the B/C/P process inspired by hidden FGPPs To demonstrate the synthetic application of this advanced B/C/P strategy inspired by FGPPs, we selected the Lycopodium alkaloid as a model. The Lycopodium alkaloids, consisting of over 200 isolated members with various architectures, have exhibited impressive biological activities [35] , [36] . Among these alkaloids, huperzine A, with particularly potent acetylcholinesterase inhibitory activity, has been used for the treatment of neurodegenerative disorders [37] , and Serratezomine A showed cytotoxicity against murine lymphoma L1210 cells (IC 50 =9.7 μg ml −1 ) and human epidermoid carcinoma KB cells (IC 50 >10 μg ml −1 ) (ref. 38 ). Because of their fascinating structures and promising biological activities, the Lycopodium alkaloids are the targets of a number of synthetic chemists engaged in total syntheses [39] , [40] . Recently, Lycopodium alkaloids lyconadins A and C were synthesized in a divergent manner using functional group pairing strategy [41] . Eight representative fawcettimine class alkaloids with different skeletons are displayed in Fig. 2 , namely lycojapodine A [42] , Serratezomine A [38] , Serratinine [43] , sieboldine A [44] , lycopladine D [45] , 8α-Hydroxyfawcettimine [46] and Lycoposerramine-S and -U [47] . In this work, we apply the aforementioned approach to the efficient and parallel syntheses of four Lycopodium alkaloids, (+)-Serratezomine A, (−)-Serratinine, (+)-8α-Hydroxyfawcettimine and (−)-Lycoposerramine-U, as well as seven complex unnatural molecules, to ultimately furnish 10 distinct polycyclic scaffolds in total. 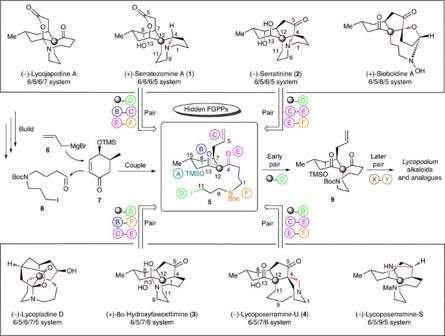Figure 2: Outline of the DOS ofLycopodiumalkaloids using the advanced B/C/P approach. Eight representative scaffolds are displayed above, and the bonds derived from their hidden FGPPs are highlighted in red. Disconnecting the pairing functional groups of Serratezomine A (1), Serratinine (2), 8α-Hydroxyfawcettimine (3) and Lycoposerramine-U (4) resulted in a common multi-functionalized precursor (5). A three-component reaction involving the assembly of building blocks (6,7and8) concisely affords the precursor (5). Through the early and later pair phases, skeletally diverseLycopodiumalkaloids and analogs may be obtained by varying functional group pairing reactions. Figure 2: Outline of the DOS of Lycopodium alkaloids using the advanced B/C/P approach. Eight representative scaffolds are displayed above, and the bonds derived from their hidden FGPPs are highlighted in red. Disconnecting the pairing functional groups of Serratezomine A ( 1 ), Serratinine ( 2 ), 8α-Hydroxyfawcettimine ( 3 ) and Lycoposerramine-U ( 4 ) resulted in a common multi-functionalized precursor ( 5 ). A three-component reaction involving the assembly of building blocks ( 6 , 7 and 8 ) concisely affords the precursor ( 5 ). Through the early and later pair phases, skeletally diverse Lycopodium alkaloids and analogs may be obtained by varying functional group pairing reactions. Full size image (+)-Serratezomine A ( 1 , 6/6/6/5 system), (−)-Serratinine ( 2 , 6/5/6/5 system), (+)-8α-Hydroxyfawcettimine ( 3 , 6/5/7/6 system) and (−)-Lycoposerramine-U ( 4 , 6/5/7/6 system) were subjected to an examination of their hidden FGPPs ( Fig. 2 ). (+)-Serratezomine A contains three FGPPs, a lactone ( B−C ), an amine ( E−F ) and an all-carbon quaternary centre ( −D , a potential pairing pattern). Similarly, (−)-Serratinine contains two quaternary centres ( −D , C−E , E−F ). (+)-8α-Hydroxyfawcettimine bears a hemiaminal ( B−F ), an α-substituted cycloketone ( C−E ) and an all-carbon quaternary centre ( −D ); (−)-Lycoposerramine-U has an additional methylene unit to connect C4 with N ( E−F ), as well as two all-carbon quaternary centres ( −D , C−E ). When disconnecting these pairing functional groups, we simplified these four natural products into a multi-functionalized precursor ( 5 ), composed of a single six-membered ring bearing two side chains that can be assembled by a three-component Michael-aldol sequence using allylmagnesium bromide 6 , enone 7 and aldehyde 8 , followed by a conventional oxidation. In the pair phase, recombining the functional groups of precursor 5 in various pairing pathways will furnish distinct Lycopodium alkaloid or alkaloid-like skeletons. Our devised early pair phase was aimed at the construction of the C11 − C12 bond utilizing the leaving group ( D ) and the active carbon centre ( ) to afford intermediate 9 . Then, the later pair phase was mainly focused on three different types of reactions, lactonization, intramolecular benzoin reaction and transannular amination, to fully manipulate the other five functional groups in 5 . Build and couple phases The allylmagnesium bromide 6 was commercially available. The enone 7 and aldehyde 8 were synthesized from known compounds in one and two steps, respectively (see Supplementary Methods for details). Notably, as emphasized by Bräse and co-workers [48] , the chiral non-racemic enone 7 may serve as a key building block for many natural products. However, its preparation was quite difficult. Accordingly, we developed an efficient new route to access the optically active enone 7 (see Supplementary Methods ). With the three building blocks in hand, we next concentrated on their coupling through a conjugate addition/aldol cascade [49] , [50] in the build phase ( Fig. 3a ). Enone 7 reacted with the freshly generated allyl cuprate prepared from 6 and then with aldehyde 8 to yield an alcohol, which, without isolation, was subsequently oxidized by Dess–Martin periodinane to produce 10 , the enol form of multi-functionalized precursor 5 , in 44% yield for two steps. Interestingly, silica gel drove the equilibrium from the 1,3-diketone to the hydrogen bond-stabilized β-keto enol 10 during purification. The precursor 10 could function equally to 5 in the pair phase as we designed in Fig. 2 . 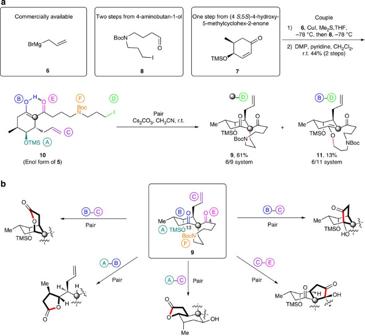Figure 3: Couple and early pair phases to prepare intermediate9. (a) Rapid access to precursor10in the couple phase and to bicyclic compounds9and11after the first pairing reaction. (b) The later pair phase was designed to rely on the formation of three lactones and two α-ketols. Figure 3: Couple and early pair phases to prepare intermediate 9 . ( a ) Rapid access to precursor 10 in the couple phase and to bicyclic compounds 9 and 11 after the first pairing reaction. ( b ) The later pair phase was designed to rely on the formation of three lactones and two α-ketols. Full size image Early pair phase We then turned to the planned early pair phase to perform the intramolecular alkylation by pairing the enol and iodide of 10 ( Fig. 3a ). Initial studies showed that, when functional group A was a t -butyldiphenylsilyl-protected alcohol, only O-alkylation occurred to yield the B−D pair, most likely due to the steric hindrance of the bulky silyl group. After we substituted the protecting group with a smaller trimethylsilyl (TMS) group, treatment of 10 with Cs 2 CO 3 in acetonitrile afforded predominantly the C-alkylation product 9 in 61% yield, as well as the O-alkylation byproduct 11 in only 13% yield. Thus, the −D pair and the B−D pair were simultaneously realized to afford a 6/9 and a 6/11 bicyclic ring systems, respectively. The highly stereoselective C-alkylation reaction may be controlled by the steric effect of the axial allylic group. Later pair phase Further pairing reactions were carried out using spirocyclic intermediate 9 . Because five functional groups ( A – C , E and F ) were present, many combinations were possible. Five pairing combinations were initially conceived between A – C and E ( Fig. 3b ), and the nucleophilic amine group F was used as the last pairing group. Pairing between A , B and C may lead to three lactones, when C is converted to a carboxyl group. Alternatively, B−C and C−E may be paired through an intramolecular benzoin reaction to form two types of α-ketols, when C is transformed to an aldehyde moiety. Lactonizations between A , B and C were first examined ( Fig. 4a ). Selective reduction of the carbonyl group at C13 in 9 with NaBH 4 in methanol [50] , followed by Lemieux–Johnson oxidation of the terminal alkene with OsO 4 /NaIO 4 (ref. 51 ) and subsequent Pinnick oxidation afforded acid 12 in high yield (83% for three steps). At this point, modifications of B to an axial hydroxyl group and C to a carboxyl group were efficiently accomplished. Acid 12 was subjected to a key one-pot ring forming reaction in two pairings, B−C / E−F or A−C / E−F , to construct the bridged δ-lactone or fused γ-lactone-based tetracyclic architecture. The bridged δ-lactone was smoothly generated when acid 12 was treated with trifluoroacetic anhydride, and after screening a number of reaction conditions (see Supplementary Table 1 ), we found that the timing for removal of the TMS group played an important role in the subsequent transannular reductive amination and intramolecular transesterification that led to the A−C pair. In fact, trifluoroacetic acid (TFA) was effective for removing the t -butoxylcarbonyl (Boc) group but only mildly effective for removing the TMS group of the δ-lactone 16 ; therefore, HCl or HF was applied to accelerate this deprotection. However, on addition of NaBH 3 CN, the transesterification product γ-lactone 14 (ref. 52 ) was primarily formed. In the absence of these inorganic acids, (+)-Serratezomine A was successfully obtained in 30% yield with its 4-epimer 13 in 19% yield, and the amount of γ-lactone 14 significantly decreased (15% yield). The configuration at C4 in 13 was confirmed by NOE analysis. 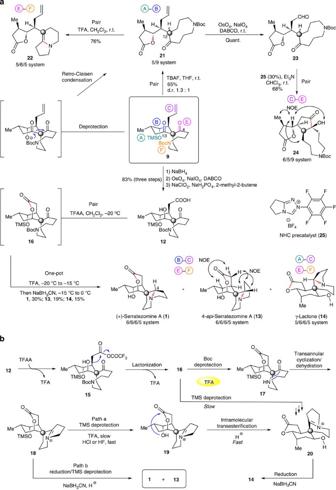Figure 4: Three lactonization-based pairing pathways. (a) Synthetic process for the concise construction of three lactones. The acid12obtained from intermediate9underwent a one-pot ring forming reaction, leading to two δ-lactones, Serratezomine A (1) and 4-epi-Serratezomine A (13) and a γ-lactone (14). A tandem deprotection/retro-Claisen condensation formed a γ-lactone, and subsequent pairing reactions efficiently afforded two tricyclic molecules (22and24). (b) Proposed mechanism for the one-pot ring forming reaction. DABCO, 1,4-diazabicyclo[2.2.2]octane. Figure 4: Three lactonization-based pairing pathways. ( a ) Synthetic process for the concise construction of three lactones. The acid 12 obtained from intermediate 9 underwent a one-pot ring forming reaction, leading to two δ-lactones, Serratezomine A ( 1 ) and 4- epi -Serratezomine A ( 13 ) and a γ-lactone ( 14 ). A tandem deprotection/retro-Claisen condensation formed a γ-lactone, and subsequent pairing reactions efficiently afforded two tricyclic molecules ( 22 and 24 ). ( b ) Proposed mechanism for the one-pot ring forming reaction. DABCO, 1,4-diazabicyclo[2.2.2]octane. Full size image On the basis of our experimental results and those reported by Kobayashi and Morita [52] , plausible reaction pathways were proposed. As depicted in Fig. 4b , on treatment with trifluoroacetic anhydride, the acid 12 was transformed to the mixed anhydride 15 , which was δ-lactonized with the axial hydroxyl group at C13. Then, both added and released TFA had the combined effect of removing the N-Boc group, but not the TMS group, in 16 , affording the free amine 17 , followed by a sequence of transannular cyclization/dehydration reactions to provide intermediate 18 . Two pathways were involved in the later reduction of iminium cation 18 : (a) When in the presence of a mineral acid (HCl or HF), the TMS group of 18 was readily removed and subsequent fast γ-lactonization via an intramolecular transesterification in 19 furnished another iminium cation ( 20 ) with a different scaffold, which was exposed to NaBH 3 CN to generate γ-lactone 14 . In this pathway, removal of the TMS group was enforced earlier, triggering the transesterification under the acidic condition. (b) Alternatively, deprotection of the TMS group in 18 with TFA was slower. Thus, when NaBH 3 CN was added, 18 was directly reduced. As a result, after removal of the TMS group, 1 and 13 were generated in a ratio of ca . 1.6:1. Conceivably, only a small portion of 18 that reacted as in ‘path a’ might undergo transesterification to produce 14 . Through this cascade process, Serratezomine A ( 1 ) and two other complex molecules containing tetracyclic skeletons ( 13 , 14 ) were efficiently synthesized in one pot. Then, our focus shifted to the other type of lactonization based on the A−B pair ( Fig. 4a ). When spirocyclic intermediate 9 was treated with tetra- n -butylammonium fluoride in tetrahydrofuran, a tandem deprotection/retro-Claisen condensation occurred to generate γ-lactone 21 in an inconsequential diastereomeric mixture (65%, d.r. 1.3:1). Further, the E−F pair was obtained through removal of N-Boc using TFA in CH 2 Cl 2 and by a subsequent transannular cyclization to afford a 5/6/5 ring system ( 22 ) in good yield (76%). We next explored another pairing pathway, between C and E . Compound 21 was converted into aldehyde 23 in quantitative yield, which was subjected to an intramolecular benzoin reaction to afford α-hydroxy ketone 24 (6/5/9 system) with Rovis’s NHC (N-heterocyclic carbene) precatalyst 25 (ref. 53 ). Next, we envisioned the intramolecular benzoin reaction to pair B−C and C−E concurrently ( Fig. 5 ). The terminal alkene in intermediate 9 was modified to an aldehyde to generate 26 , which was subjected to the intended benzoin reaction. After screening different bases, solvents and temperatures (see Supplementary Table 2 ), we found that, on treatment of 26 with NHC precatalyst 25 and triethylamine in chloroform at 55 °C, 27 and 28 were successfully produced in 51 and 42% isolated yields, respectively. The structures of 27 and 28 were confirmed by two-dimensional NMR spectra. Further functional group pairings were performed based on these two tricyclic molecules. A one-pot deprotection/transannular N-alkylation of 27 afforded a 6/5/6/5 system ( 29 ) in good yield (62%), which completed the E−F pair. An X-ray analysis of 29 confirmed its relative configuration. Then, we further explored the feasibility of pairing the two ketone moieties ( C−E ) in 27 . Inspired by the pyrrolidine ring of Lycoposerramine-S, we exposed 27 to methylamine hydrochloride and sodium cyanoborohydride [54] , resulting in stereoselective double reductive aminations to afford compound 30 with a 6/5/5/9 skeleton in good yield (65%, 77% brsm). The stereochemistry of 30 was unambiguously confirmed by NOE analysis. 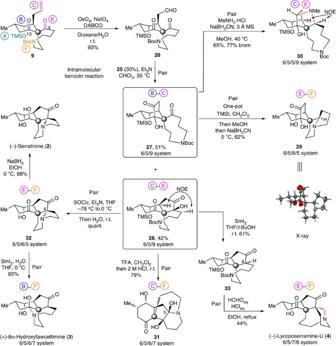Figure 5: Divergent pairing pathways to six complex tetracyclic scaffolds. Intramolecular benzoin reaction of aldehyde26obtained from intermediate9afforded two α-ketols (27and28). Starting from27and28, Serratinine (2), 8α-Hydroxyfawcettimine (3) Lycoposerramine-U (4) and three different tetracyclic scaffolds were readily produced through selective functional group pairing reactions within one to two steps. Figure 5: Divergent pairing pathways to six complex tetracyclic scaffolds. Intramolecular benzoin reaction of aldehyde 26 obtained from intermediate 9 afforded two α-ketols ( 27 and 28 ). Starting from 27 and 28 , Serratinine ( 2 ), 8α-Hydroxyfawcettimine ( 3 ) Lycoposerramine-U ( 4 ) and three different tetracyclic scaffolds were readily produced through selective functional group pairing reactions within one to two steps. Full size image Meanwhile, α-ketol 28 was used for the following pairing reactions. The C−F pair was first investigated. After removal of the Boc group with TFA, the carbinolamine was produced at C5 exclusively [55] . Subsequent TMS deprotection gave 31 as a tetracyclic system (6/5/6/7) in 79% yield. Moreover, the E−F pair was efficiently constructed through an intramolecular S N 2 reaction when 28 was treated with SOCl 2 and Et 3 N in tetrahydrofuran [50] . Compound 32 was obtained on removal of the TMS group by in situ -generated acid to afford the same 6/5/6/5 framework as in ( − )-Serratinine ( 2 ). Selective reduction of 32 with sodium borohydride in anhydrous ethanol [55] afforded ( − )- 2 in excellent yield (88%). Gratifyingly, (+)-8α-Hydroxyfawcettimine ( 3 ) was also synthesized from 32 via reductive cleavage of the C4–N bond, followed by carbinoamine formation using SmI 2 (ref. 50 ). In addition, the B−F pairing (as a carbinoamine) in place of the C−F pairing was performed to exclusively furnish (+)- 3 with a 6/5/7/6 ring system. Ultimately, we focused on the synthesis of the (−)-Lycoposerramine-U ( 4 ) skeleton (6/5/7/6). SmI 2 reduction of α-ketol 28 successfully afforded diketone 33 as an inseparable mixture of two C4 epimers. A tandem deprotection/transannular Mannich reaction of diketone 33 using dilute aqueous HCl and formaldehyde [56] afforded the tetracyclic (−)-Lycoposerramine-U ( 4 ) in moderate yield (44%), completing the E−F pair. In this work, we have introduced an advanced B/C/P strategy for the DOS of natural products and natural product-like molecules that is inspired by FGPPs. In this process, identifying the FGPPs of these natural molecules is key, and the following recombination of functional groups should significantly increase the diversity of comparably complex scaffolds and decrease the total steps needed for the synthesis of these unnatural analogues as well. The build and couple phases are designed to allow the generation of a unified precursor containing at least the required functional groups that existed in the natural products. The Lycopodium alkaloids were selected for a demonstration of this advanced B/C/P strategy. Extensively utilizing the functional groups within the unified precursor 5 , we efficiently synthesized 10 distinct complex skeletons through various functional group pairing pathways ( Fig. 6 ). All syntheses were accomplished within seven to nine steps from 4-aminobutan-1-ol, providing 2–16 mg of each final product, sufficient for characterizations and most biological assays. Remarkably, four natural alkaloids were obtained in this concise and parallel process, in particular, the shorter total synthesis of (+)-Serratezomine A [57] , the first asymmetric total synthesis of (−)-Serratinine [58] and the first total syntheses of (+)-8α-Hydroxyfawcettimine and (−)-Lycoposerramine-U. Moreover, six other complex and diverse natural product-like scaffolds were also efficiently furnished, which further demonstrated the capability of this FGPP-inspired B/C/P strategy for the generation of a novel chemical library to probe chemical space. We expect that this new strategy will be applied both to other complex natural products possessing FGPPs and to generating natural product-like chemical libraries of skeletally complex and diverse molecules for chemical genetics and drug discovery. 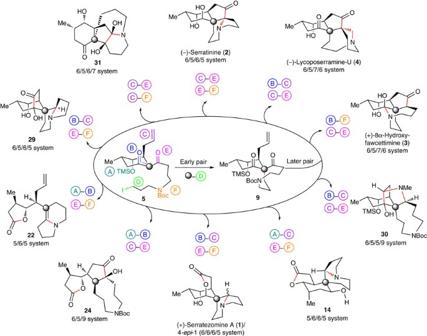Figure 6: Full list of the final natural and unnatural scaffolds. In total, 11 polycyclic molecules containing 10 distinct skeletons were obtained from precursor5through the early and later pair phases. The formed bonds from FGPPs are highlighted in red. Figure 6: Full list of the final natural and unnatural scaffolds. In total, 11 polycyclic molecules containing 10 distinct skeletons were obtained from precursor 5 through the early and later pair phases. The formed bonds from FGPPs are highlighted in red. Full size image General analytic methods 1 H NMR spectra were recorded on a Varian 400 MHz spectrometer at an ambient temperature with CDCl 3 or CD 3 OD as the solvent unless otherwise stated. 13 C NMR spectra were recorded on a Varian 100 MHz spectrometer (with complete proton decoupling) at an ambient temperature. Chemical shifts are reported in parts per million relative to CDCl 3 or CD 3 OD ( 1 H, δ 7.26 for CDCl 3 , 3.31 for CD 3 OD; 13 C, δ 77.00 for CDCl 3 , 49.00 for CD 3 OD). Data for 1 H NMR are reported as follows: chemical shift (p.p.m. ), integration, multiplicity (s=singlet, d=doublet, t=triplet, q=quartet, m=multiplet and br=broad) and coupling constants (Hz). Infrared spectra were recorded on a Thermo Fisher FT-IR200 spectrophotometer. High-resolution mass spectra were recorded at Peking University Mass Spectrometry Laboratory using a Bruker Apex IV FTMS spectromete. Circular dichroism (CD) spectra were measured on an Applied Photophysics π*-180 spectrometer. Preparative HPLC-MS on a Waters Auto Purification LC/MS system (3100 Mass Detector, 2545 Binary Gradient Module, 515 HPLC pump, 2767 Sample Manager and 2998 Photodiode Array Detector). The system was equipped with a Waters C18 5 μm X-bridge separation column (150*4.6 mm). Optical rotations were recorded on an AUTOPOL III digital polaimeter at 589 nm and are recorded as (concentration in grams per 100 ml solvent). Analytical thin layer chromatography was performed using 0.25 mm silica gel 60-F plates. Flash chromatography was performed using 200–400 mesh silica gel. Materials All reagents were used as supplied by Sigma-Aldrich, J&K and Alfa Aesar Chemicals. Methylene chloride, acetonitrile and dimethyl formamide were distilled from calcium hydride; chloroform was distilled from anhydrous potassium carbonate; tetrahydrofuran, diethyl ether and 1,4-dioxane were distilled from sodium/benzophenone ketyl before use. All reactions were carried out in oven-dried glassware under an argon atmosphere unless otherwise noted. Chemical synthesis All syntheses were carried out according to Supplementary Methods . NMR spectra of the compounds involved in this study were shown in Supplementary Figs 1–63 . For CD spectra of compound 3 and 4 , see Supplementary Figs 64–65 . NMR data and [α] D or CD data comparisons of natural and synthetic products ( 1 – 4 ) were displayed in Supplementary Tables 3–10 . X-ray crystallographic image and data of compound 29 were displayed in Supplementary Fig. 66 and Supplementary Tables 11 . Accession codes: The X-ray crystallographic coordinates for structures reported in this article have been deposited at the Cambridge Crystallographic Data Center, under deposition number CCDC 988148. These data can be obtained free of charge from the Cambridge Crystallographic Data Centre via www.ccdc.cam.ac.uk/data_request/cif . How to cite this article : Zhang, J. et al. Diversity-oriented synthesis of Lycopodium alkaloids inspired by the hidden functional group pairing pattern. Nat. Commun. 5:4614 doi: 10.1038/ncomms5614 (2014).